Requirements for fault-tolerant factoring on an atom-optics quantum computer Quantum information processing and its associated technologies have reached a pivotal stage in their development, with many experiments having established the basic building blocks. Moving forward, the challenge is to scale up to larger machines capable of performing computational tasks not possible today. This raises questions that need to be urgently addressed, such as what resources these machines will consume and how large will they be. Here we estimate the resources required to execute Shor’s factoring algorithm on an atom-optics quantum computer architecture. We determine the runtime and size of the computer as a function of the problem size and physical error rate. Our results suggest that once the physical error rate is low enough to allow quantum error correction, optimization to reduce resources and increase performance will come mostly from integrating algorithms and circuits within the error correction environment, rather than from improving the physical hardware. The prospect of an entirely new industry based on quantum mechanics has motivated technological development and led to a much better understanding of the principals governing our universe at the atomic scale. For quantum technology, experimental progress has been pronounced [1] , [2] , [3] , [4] , [5] , [6] . Not only has a fledgling industry based on quantum key distribution emerged [7] , [8] , but many experimental groups now routinely demonstrate the creation, manipulation and measurement of multiple qubits in various physical systems with increasingly higher accuracy [9] . The goal of developing a viable, large-scale quantum computer is now in sight, due in part to recent theoretical progress. Techniques for fault-tolerant quantum error correction, necessary to deal with imperfect physical components, have been substantially refined [10] , [11] , [12] . Adaptation of these techniques to the physical restrictions of quantum hardware has led to multiple architecture designs, each one representing a pathway towards a future quantum computer [13] , [14] , [15] , [16] , [17] , [18] , [19] , [20] , [21] . Although a large-scale quantum computer is still years away, it is now possible to make qualitative and quantitative predictions about the performance and required hardware resources for such a computer. Some estimates consider architectures based on specific physical systems [20] , [21] , [22] , [23] , [24] , an essential aspect in resource analysis. However, these estimates omit a full prescription for executing the algorithms in question. Others consider promising error-correction codes and circuits, such as post-selection [10] and topological models [12] , yet do so without reference to particular architectures or applications. Above the physical device level, there are a number of implementation layers required to reliably execute a quantum algorithm. By careful choice of all technological elements and the integration of all implementation layers, a complete analysis is now possible. A full account of the resources required for fault-tolerant quantum computation must consider several factors. Because physical components will fail and introduce errors, an error-correction code must be chosen and then adapted to any restrictions imposed by the hardware. Physical error rates must be suppressed below the fault-tolerant threshold of the chosen code. Next, the code restricts the set of logical gates that can be directly applied to encoded data. Each gate in the high-level quantum algorithm must be decomposed into a universal set of fault-tolerant primitives. To realize these universal primitives, ancillary states and protocols are typically required to enact teleported gates that could otherwise not be directly applied to the encoded data [25] . Each of these steps increases the total qubit/time overhead and must be carefully integrated in a way that ensures all steps are counted. The precise details of how resources are calculated depend on the properties of the architecture in question, the techniques used for fault-tolerant error correction and the circuit-based description of the desired algorithm. One of the most promising error correction techniques is topological error correction; defined over a large three-dimensional cluster state of qubits [12] . This error correction technique, despite the fact that it is well suited to large-scale architectures, has only briefly been studied in regards to how a large-scale algorithm will actually be implemented. In a scalable quantum computer, high-level quantum programming languages will be required to control quantum algorithms [26] , [27] , [28] , [29] , and effective methods will be required to synthesize logical circuits for these algorithms [30] , [31] , [32] . Logical circuits will need to be compiled to a restricted set of fault-tolerant operations available in the topological model. Finally, circuits will need to be expressed in terms of physical operations in the quantum computer—in the topological model, this requires the construction of compact braided logic. These steps have a direct impact on the physical resources needed for computation, and a concerted effort to understand these requirements has only just begun [33] . Typically, estimates consider the number of required gates in the high-level quantum algorithm and the basic amount of ancillary space needed for additional fault-tolerant protocols [20] , [21] , [22] . However, these estimates provide only a partial analysis. Error correction codes inevitably suffer from constraints that need to be taken into account; for example, the interaction of qubits required by the actual algorithm with qubits needed for ancillary protocols. The scheduling and routing of these ancillary protocols are often overlooked when estimating resources and are likely to dramatically affect the resource estimates [34] , [35] . The compatibility of the topological model with hardware architectures has been demonstrated in Devitt et al. [18] , Yao et al. [19] , Meter et al. [20] Jones et al. [21] In our complete analysis, we consider an atom-optics architecture [18] , [36] , based on the photonic module [37] . The photonic module is a relatively simple device that allows an atomic qubit to mediate the generation of photonic entanglement. The three-dimensional cluster state that supports topological error correction is created by an array of these devices. Decomposition of each logical gate into a series of physical operations in this architecture is straightforward, and hence all geometry and connectivity constraints at both logical and physical levels can be explicitly included in the analysis. The desired algorithm, Shor’s algorithm, is a comparatively simple application compared with other problems solvable by a quantum computer [24] , [38] . More importantly, it has a rich history of theoretical development and a number of explicit circuit constructions [39] , [40] , [41] . In the present study, we begin with a suitable circuit from the literature and further compile the circuit to one that is fault-tolerant and error corrected. We choose an explicit construction amenable to the system design described above. However, to run the circuit, we still have to take the geometric constraints at the logical level into account. Even though scheduling at the physical level is taken care of by the topological model, scheduling and arrangement of gates and ancillary operations within the logical space impacts performance. This step is largely unexplored and leaves substantial room for optimization. The ability of an error-corrected computer to achieve the optimal circuit size at the logical level is dependent on adapting to these constraints, hence estimates should be made with care. Our results show that factoring a 1,024-bit number requires ~2.3 years of computational time and ~1.9 billion quantum devices. These resources are higher than other estimates; however, the numbers are an accurate reflection of the quantum circuit and the error correction model. Our results illustrate that the sophisticated techniques in quantum compilation must be developed and that these techniques can significantly reduce the resources required to execute large-scale quantum algorithms. Preliminaries In the topological cluster state model, a three-dimensional cluster forms the effective Hilbert space in which computation takes place [12] , [42] . In the architecture, a photonic cluster state is continuously prepared from non-entangled photons by the hardware. Logical qubits are introduced as pairs of defects in the cluster. Defects are created in the cluster by measuring physical qubits in the Z- basis [12] . An entangling gate is realised by braiding pairs of defects. Logical errors occur when chains of physical errors connect or encircle defects, which is made less likely by increasing the circumference of defects and by increasing their separation. Physical qubits in the bulk of the cluster, those not associated with defects, are measured in the X -basis. These measurements reveal the endpoints of chains of errors, from which the most likely set of errors can be inferred. To estimate physical resources, we are ultimately interested in the size of the three-dimensional cluster state required to execute Shor's algorithm. As the algorithm is executed at the logical level, it is useful to introduce a scale factor that essentially encapsulates the overhead associated with error correction [12] . A logical cell is defined as a three-dimensional volume of the cluster that has an edge length of d + d /4 unit cells, where d is the distance of the error-correction code. Defects have circumference of d unit cells and are separated by d unit cells (illustrated in Fig. 1 ). 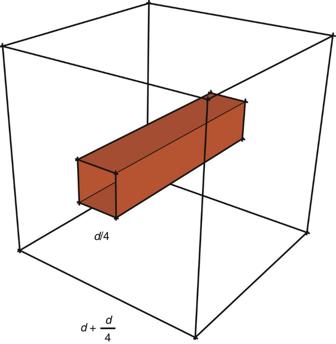Figure 1: A logical cell. The size of topological quantum circuits are expressed in terms of logical cells, giving an error correction-independent measure. The lengths are expressed in terms of unit cells of the cluster state. The defect is the coloured region within the cell. Pairs of defects form a logical qubit. Figure 1: A logical cell. The size of topological quantum circuits are expressed in terms of logical cells, giving an error correction-independent measure. The lengths are expressed in terms of unit cells of the cluster state. The defect is the coloured region within the cell. Pairs of defects form a logical qubit. Full size image Shor’s algorithm There are a number of different circuit implementations for this algorithm [39] , [40] , [41] , which assume that arbitrary sets of qubits can be simultaneously entangled without any penalty related to their separation. This is not the case in the topological model, as gates are realised by braiding defects, which occupy physical space in the cluster. The scheduling required to implement multiple gates over long distances in the same time step is non-trivial and will likely add significant overhead. A simpler approach is to use a circuit that has already been modified to require only nearest neighbour gates in some restricted geometry. We have chosen to use the Beauregard circuit, which is a linear nearest neighbour (LNN) construction with swap gates used to rearrange qubits in the circuit [43] , [44] . This circuit is not as efficient as others, but its explicit LNN construction means it can be applied in the topological model without modification. The Beauregard circuit performs modular exponentiation in Fourier space, which is usually approximated, while modular exponentiation based on reversible Boolean circuits is exact [45] . However, the complicated nature of fault-tolerant protocols makes the manual design and optimization of Boolean addition intractable. With logical qubits arranged in a line, the circuit to factor an L -bit number requires Q =2 L qubits and has depth K =32 L 3 to the leading order. The circuit is not inherently robust to errors [46] , requiring an error rate per gate ~ 10 −1 / KQ =10 −1 /64 L 4 to ensure a 90% chance of success. Topological circuits The Methods section details the steps that decompose Shor’s algorithm into a valid set of operations that can be performed in the topological model. We can translate this decomposed circuit into a sequence of braids (a topological circuit) in the three-dimensional cluster state. In the Methods section, we detail the geometric structures of all the valid topological operations; initialization, measurement, state injection, teleportation and the CNOT gate. Decomposing Shor’s algorithm with respect to these gates converts the algorithm into a sequence of R z ( π /8) rotations, which dominate the resource costs of the algorithm. This is the logical gate that will be designed. Shown in Fig. 2 is the topological circuit for the logical R z ( π /8) rotations with one and two levels of concatenated state distillation. The full details underlying the topological circuit in Fig. 2 can be found in Supplementary Figs S1–S8 and the Supplementary Discussion . The topological circuits are compressed manually into cuboids such that they can be stacked tightly in both the spatial and temporal directions in the cluster. The algorithmic qubits (the qubits specified in the Beauregard circuit) are the defects marked as green (two defects per algorithmic qubit occupying a cross-sectional area of two logical cells). Immediately above each algorithmic qubit is an empty region of the cluster—this space is used for CNOT gates needed in the Beauregard circuit and swap gates required by the Beauregard circuit. Because the layout of algorithmic qubits in the cluster mimics the LNN aspect of the Beauregard circuit, no optimization is required to achieve the original circuit depth. Above the empty region is the distillation space for | Y › states, required to implement a R z ( π /4) correction for each applied R z ( π /8) gate and for Hadamard operations. Below the algorithmic qubits is the distillation space for | A › states, Fig. 3 illustrates. 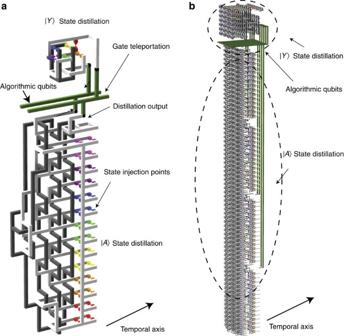Figure 2: Topological circuits for aRz(π/8) rotation in the topological cluster. Panelashows one level of concatenated state distillation, whereas panelbis for two levels. The temporal axis in the cluster is illustrated. For a detailed explanation of these constructions seeSupplementary Figs S3–S8and theSupplementary Discussion. Qubits that are part of the algorithmic circuit for Shor's algorithm are illustrated in green and represent a small fraction of the total circuit. The white and dark structures represent primal and dual defects in the topological cluster whereas the coloured pyramids are injection points corresponding to the circuit elements illustrated inSupplementary Fig. S2. The volumes and depths of these two circuits areV={210,1386} andD={5,9} logical cells, respectively. Figure 2: Topological circuits for a R z ( π /8) rotation in the topological cluster. Panel a shows one level of concatenated state distillation, whereas panel b is for two levels. The temporal axis in the cluster is illustrated. For a detailed explanation of these constructions see Supplementary Figs S3–S8 and the Supplementary Discussion . Qubits that are part of the algorithmic circuit for Shor's algorithm are illustrated in green and represent a small fraction of the total circuit. The white and dark structures represent primal and dual defects in the topological cluster whereas the coloured pyramids are injection points corresponding to the circuit elements illustrated in Supplementary Fig. S2 . The volumes and depths of these two circuits are V ={210,1386} and D ={5,9} logical cells, respectively. 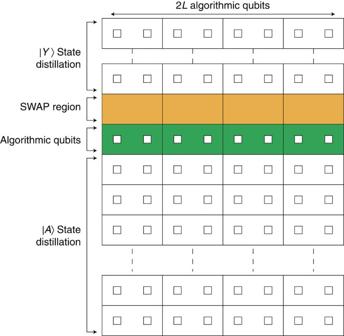Figure 3: Layout of logical qubits for Shor's algorithm. The layout includes the necessary cluster space for |A› and |Y› state distillation. The small squares represent the defects that exist within each larger box defining a cross-sectional area of a logically encoded qubit. The region for algorithmic qubits is green, a SWAP region for performing gates between algorithmic qubits does not contain any defects and is illustrated in orange whereas the regions devoted to state distillation are illustrated in white. Full size image Figure 3: Layout of logical qubits for Shor's algorithm. The layout includes the necessary cluster space for | A › and | Y › state distillation. The small squares represent the defects that exist within each larger box defining a cross-sectional area of a logically encoded qubit. The region for algorithmic qubits is green, a SWAP region for performing gates between algorithmic qubits does not contain any defects and is illustrated in orange whereas the regions devoted to state distillation are illustrated in white. Full size image At one level of concatenation, each algorithmic qubit has a dedicated | A › and | Y › state distillery. As the algorithmic layer is linear, these distilleries connect from above and below in the cluster, where direct connections in the topological model correspond to teleported gates [12] . At two levels of concatenation, the topological circuit encapsulates four algorithmic qubits. The first concatenation level has physical injection points for low fidelity | A › and | Y › states, and the size of the defects is half of what is required at the algorithmic layer. This reduction in size and separation of defects for the first concatenation level reflects the fact that distillation circuits have a residual error. If the error of an injected state at the physical level is O (10 −3 –10 −4 ), then implementing full-strength error correction for these circuits is redundant, as the residual error from distillation will always dominate. At the second layer of concatenation, the residual error becomes commensurate with the required logical error needed for computation. Therefore, after the first layer of concatenation, defects are expanded and separated to the same size and distance as in the required error correction for the algorithm. Additionally, at the second level of the | A › state distillation circuit, we require the distilled | Y › state at the first level of concatenation. The appropriate circuits are placed in the relevant free space in the cluster, as required. The application of corrective R z ( π /4) rotations for | A › state distillation and the probabilistic nature of the circuits themselves are compensated for at the second level of concatenation by placing extra distilleries in the cluster (see the Supplementary Discussion section). For | Y › state distillation, there is sufficient space for one extra circuit adjacent to the second-level circuit, to compensate for any one failure at level one. For | A › state distillation, there is space for two extra circuits within the cuboid to compensate for a given circuit failure. These circuit failures occur with probability of O ( p ), where p is the error associated with the injected states. Given the additional level one circuits that we have incorporated into the gate and assuming p is of O (10 −3 –10 −4 ), we will have too many failures at level one with a probability of O (10 −5 –10 −7 ) for | Y › states and of O (10 −7 –10 −9 ) for | A › states, respectively. Therefore, we expect that we will not have sufficient first-level states every 10 5 –10 7 logical gates. Although these failures lead to an increase in circuit depth, they occur infrequently enough to be neglected. Finally, at the second level of state distillation, a total of 15 first-level circuits for corrective | Y › states, needed by the second-level | A › state circuit, are used. The probability that not enough level-one | Y › states are available is given by 15 p /2 15 . This occurs when all 15 R z ( π /8) corrections are needed, and a single level-one | Y › distillation failure occurs, and if p is of O (10 −3 ), this is also of O (10 −7 ). Corrective | Y › states, needed with a probability of 0.5, for the logical R z ( π /8) gate are located above the algorithmic layer. The total logical volume of cluster for one and two levels of state distillation can be calculated explicitly. For one level of concatenation, each R z ( π /8) gate occupies a volume of V =5 × 21 × 2 cells with a depth along the temporal axis of the cluster of D =5 cells and a cross-sectional area of A =21 × 2. For two levels of concatenation, the volume is V =8 × 77 × 9/4 with a depth along the temporal axis of D =9 and a cross-sectional area of A =77 × 2/4. The factor of 1/4 accounts for the fact that the cuboid represents four gates. Cluster volume To determine the total size of the cluster state, we need to know the amount of error correction and state distillation required. Each logical gate requires Λ × V logical cells. The factor of Λ comes from the decomposition of each gate at the algorithmic level into R z ( π /8) gates [47] . This decomposition is detailed in the Methods section. Hence, the failure probability of such a gate needs to be where p f is the failure rate of a logical cell. The right hand side sets the target failure rate for the logical gates in the circuit for Shor’s algorithm. For standard depolarizing noise, we can estimate the failure probability of a single logical volume of the cluster as p f ≈ C 1 ( C 2 p / p th ) ⌊ ( d +1)/2 ⌋ , where d is the distance of the code, p is the physical error rate, p th is the threshold error rate (≈0.62%), C 1 ≈0.13, and C 2 ≈0.61 (ref. 12 ). Assuming that p f <<1 and 1/640 L 4 <<1, the distance required to achieve the target error rate is Here we use the fact that the residual error after l levels of state distillation should be below the error rate of a logical cell, such that 35 ( 3 l − 1 ) / 2 p 3 l ≤ p f and 35 ( 3 l − 1 ) / 2 p 3 l ≤ p f for | Y › states | A › states, respectively. These conditions determine the level of state distillation required. Only for very large L ( L ≳ 2 16 ) or for high values of P ( ≳ 0.001) does state distillation require three levels. The volume and depth at this level was extrapolated from the level-two circuits to be V =10,000 and D =15. Finally, we can specify the properties of the entire cluster state. The cluster contains 4 L × A logical cells. The total cross-sectional area of the cluster is 5 Ld × 5 dA /4 physical unit cells. The third dimension of the cluster represents the temporal axis, and its length determines the computational time. The depth of a single logical gate is Λ × D , and the depth of a single R z ( π /8) gate is Λ D × (5 d /4). Therefore, the total depth of the cluster is (32 L 3 Λ D ) × (5 d /4). Physical resources In the architecture, photonic modules are used to prepare the cluster state as well as to initialize and measure single photons [36] . There is a one-to-one mapping between the cross-sectional size of the three-dimensional cluster and the number of required modules. For a cluster with a cross-sectional area of N 1 × N 2 physical unit cells, a total of (2 N 1 +1)(2 N 2 +1) optical lines exist. Of these, (2 N 1 +1)(2 N 2 +1)/2 lines require two modules for photon detection and (2 N 1 +1)(2 N 2 +1)/2 lines require four modules. All optical lines require one module as a probabilistic photon source. The number of modules required to prepare the cluster state is 2( N 1 +2)( N 2 +1)+2( N 2 +2)( N 1 +1) [18] . This gives a total number of modules equal to (12+14 N 1 +14 N 2 +20 N 1 N 2 ), where N 1 =5 Ld and N 2 =5 d /4 A . In addition to the number of modules, we can specify the physical size of the computer and its runtime. The dimensions of the computer are S x =5 LdM and S y =5 dMA /4, where M × M is the surface area of a photonic module (with depth< M ) [18] . The physical depth of the computer is S z ≤2 Tc f , where c f is the speed of light in fibre and T is the time required to prepare a single layer of the cluster state [18] , corresponding to the operational speed of the photonic module. This depth is governed by the optical lines that recycle photons from the detectors to the sources [36] . The time required to run the algorithm is 32 L 3 Λ D × 5 d /4 × 2 T . 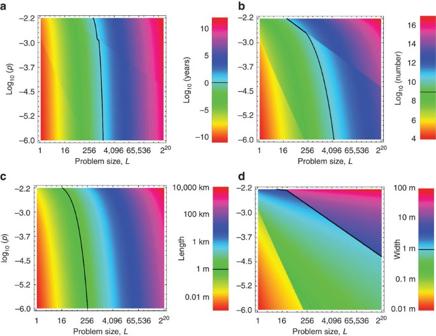Figure 4: Physical resources required for factoring. Each panel illustrates the resources required to factor anL-bit number with an error ratep.Panelashows the computational time to complete factoring assuming aT=10 ns operational time for the photonic module. The solid line is where factoring takes 1 year. Panelbshows the number of photonic modules with the solid line showing where factoring requires one billion modules. Panelscanddillustrate the computer size, assuming each photonic module has a cross-sectional size of 100 × 100 μm. The solid line is when the length or width of the computer reaches 1 m. The discontinuities represent points where the concatenation level of state distillation increases. Figure 4 shows the runtime of the algorithm, the total number of photonic modules and the dimensions of the computer as functions of the physical error rate and the problem size. Here we have assumed that p th =0.62% (refs 12 , 48 ), M =100 μm and T =10 ns (ref. 49 ). Contour lines in Fig. 4 indicate when the completion time is 1 year, when the total number of photonic modules is one billion and when the cross-sectional dimensions are 1 m. With a physical error rate an order of magnitude below the threshold and without any further algorithmic improvements, the largest problem size that can be completed within a year is L ≈810. Figure 4: Physical resources required for factoring. Each panel illustrates the resources required to factor an L -bit number with an error rate p. Panel a shows the computational time to complete factoring assuming a T =10 ns operational time for the photonic module. The solid line is where factoring takes 1 year. Panel b shows the number of photonic modules with the solid line showing where factoring requires one billion modules. Panels c and d illustrate the computer size, assuming each photonic module has a cross-sectional size of 100 × 100 μm. The solid line is when the length or width of the computer reaches 1 m. The discontinuities represent points where the concatenation level of state distillation increases. Full size image A recent milestone was the factorization of a 768-bit RSA modulus over several years using the number field sieve classical factoring method [50] . Hence, these results show the clear advantage of quantum computation. They seem not to demonstrate a significant increase in the processing power of quantum computers. Our results give a comfortable upper bound for the resource requirements using explicit circuit constructions in the topological model. The time required to factor a 1024-bit number in this analysis is 2.3 years with 1.9 billion photonic modules required to prepare the cluster. An interesting question is how these numbers can be compared with the fundamental circuit used in this analysis. As we mentioned in the introduction, there are different techniques to construct a circuit for Shor's algorithm. The overhead associated with error correction should be calculated based on the resource costs associated with the same non-error-corrected circuit. For instance, the circuit using Toffoli-based quantum adders [45] and/or using an approximate quantum fourier transform [51] could reduce the overall physical recourses; however, the error correction overhead is highly non-trivial. In this analysis, the basic circuit requires a computational depth of 32 L 3 and 2 L qubits. For physical gate times of 10 ns, for L =1,024, the error correction overhead amounts to a factor of 2.3 × 10 5 in time and 9.1 × 10 5 in terms of qubits (modules). These numbers are based on a physical error rate an order of magnitude below threshold. This overhead can be significantly reduced by optimisations unrelated to the fundamental hardware. This is illustrated by the fact that decreasing the error rate by an order of magnitude results in a computational speed-up to 1.2 years. The same speed-up can be achieved by compacting the topological circuits shown here by ~ 45% along the temporal axis of the cluster. There have been several other resource estimates made for various quantum computer architectures using concatenated and topological error correction. Thaker et al. [22] estimated that to factor a 1,024-bit number on an architecture based on trapped ions would take around 25 days. Van Meter et al. [20] estimated that a 2048-bit number on a distributed architecture based on quantum dots would take around 400 days . Jones et al. [21] recently improved the latter estimate to around 10 days by using a monolithic array of dots and increasing the speed of error correction. New results in superconducting designs suggest a factoring time for a 2,000-bit number of slightly less than 1 day [52] . The differences in these estimates arise due to how the algorithm is implemented. In particular, more resource-efficient techniques are utilized in these results, which need to be explicitly integrated within the topological model. All resource estimates, including ours, illustrate that a large fraction of the overhead arises from the need to prepare ancillary states. Other results assume sufficient space within the computer such that ancillary protocols can be completed rapidly enough so that the depth of the algorithmic circuit is unchanged. This could be of significant benefit. However, the appropriate routing of these ancillary protocols needs to be explicit. How distillation circuits are interfaced with data qubits needs to be detailed, and which protocols are utilized needs to be analysed. Estimates from Jones et al. , [21] and Fowler et al. [52] use the most optimal circuit for Shor's algorithm [39] , [45] ; however, this circuit has not yet been adapted to the geometric constraints of the topological cluster. Until an appropriate construction is presented for the topological cluster, it is difficult to assume that the circuit size will remain unchanged. If such a circuit design is presented, then we anticipate immediate reductions in resources. Previous results also assume that various subcomponents of a fault-tolerant implementation can be applied without space/time penalty. There have been many results published optimizing various components in a fully error-corrected quantum algorithm [53] , [54] , [55] , [56] . However, each of these results has been derived in isolation, some have not been converted into the topological model and none have been carefully integrated together. This is the primary challenge of topological compilation. Subcomponents may be efficient, but the success of a large-scale computation requires delicate integration. Our results illustrate that there is a significant gap between optimistic resource estimates and those performed using explicit circuit constructions. It is clear that algorithmic compilation is a necessity before a quantum computer is actually built. Reducing the burden on experimental development is ultimately a function of how we realize abstract algorithms. Our results illustrate that there is still much work to be done. Although the topological model is promising, its ultimate success is dependent on continual efforts to integrate all necessary protocols in a way that minimizes the number of devices and the time required to execute an algorithm. Valid operations in the Topological cluster There are five primitive, fault-tolerant operations allowed in the topological model: measurement, initialization, state injection, the two-qubit CNOT and the teleported phase rotations . These are illustrated in Fig. 5 . There are two types of defects that can be created, primal and dual. Braided logic operations can only occur between defects of opposite type and the geometric structures for X- and Z -basis initialization and measurement are interchanged depending on the type of defect. 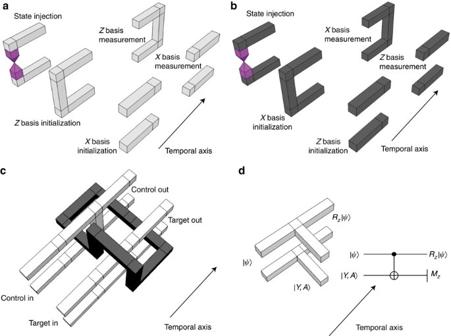Figure 5: Examples of basic operations used to construct braid sequences. (a) Primal defects (white) in a horseshoe shape are used to prepare a logical qubit in the state |0› and to measure a logical qubit in theZ-basis. An arbitrary state can be prepared by measuring one of the physical qubits (shown in pink) in a rotated basis as the defects are created. (b) Dual defects (dark) in a horseshoe shape are used to prepare a logical qubit in the state |+› and to measure a logical qubit in theX-basis. (c) A CNOT gate can be achieved by braiding a pair of dual defects (prepared in the state |+›) with three pairs of primal defects (the control qubit, the target qubit and an extra qubit prepared in the state |0›)14. (d) Teleportedrotations can be achieved by attaching the relevant ancillary state to the data qubit12. Figure 5: Examples of basic operations used to construct braid sequences. ( a ) Primal defects (white) in a horseshoe shape are used to prepare a logical qubit in the state |0› and to measure a logical qubit in the Z -basis. An arbitrary state can be prepared by measuring one of the physical qubits (shown in pink) in a rotated basis as the defects are created. ( b ) Dual defects (dark) in a horseshoe shape are used to prepare a logical qubit in the state |+› and to measure a logical qubit in the X- basis. ( c ) A CNOT gate can be achieved by braiding a pair of dual defects (prepared in the state |+›) with three pairs of primal defects (the control qubit, the target qubit and an extra qubit prepared in the state |0›) [14] . ( d ) Teleported rotations can be achieved by attaching the relevant ancillary state to the data qubit [12] . Full size image Gate decomposition As in the case of all error-corrected models of quantum computation, the topological model does not allow all gate operations to be directly applied in a fault-tolerant manner. At the logical level, only preparation of the states |+› and |0›, X and Z gates, measurement in the X and Z bases, and the CNOT gate can be directly applied. Swap gates are achieved by deforming the trajectory of the defects. To complete a universal set, we add the R z ( π /8) and R z ( π /4) rotations [12] . The R z ( π /4) rotation is constructed using the [[7,1,3]] Steane code to distil an appropriate ancillary state. This construction of the R z ( π /4) rotation is more resource efficient than two R z ( π /8) rotations, which require distillation protocols based on the [[15,1,3]] Reed–Muller code. To apply these gates, we perform a teleportation operation with the ancillary states and . Each time we attempt the R z ( π /8) gate, there is a 50% chance that a R z ( π /4) correction is required. To ensure that the error rate of the R z rotations is sufficiently low, the states | A › and | Y › must be of sufficient fidelity. As these ancillary states are prepared in the cluster via injection protocols [12] , state distillation is used to increase the fidelity of the ancilliary states [25] , consuming multiple | A › or | Y › states with a lower fidelity. This process can be concatenated until the desired fidelity is reached. If p l is the error probability of the state after l levels of state distillation, then and for | A › and | Y › states, respectively [25] . Each distillation circuit is probabilistic with a failure probability of O ( p ). Supplementary Fig. S2 illustrates the quantum circuits for these distillation protocols, and Supplementary Fig. S1 illustrates the compacted topological structures. Given our set of logical gates, which now includes the R z ( π /8) rotation, we decompose the circuit for Shor's algorithm into an appropriate sequence of these operations. To estimate an upper bound on the number of gates required, we will (pessimistically) assume every gate is a non-trivial phase rotation. These rotations must be approximated by a sequence of logical gates found using the Solovay–Kitaev algorithm [57] . ~50% of the gates in this sequence [58] are R z ( π /8) rotations, which are the most resource intensive of our logical gates. For simplicity, we will (pessimistically) assume all of these gates are R z ( π /8) rotations. Recent algorithms, which can efficiently calculate these been developed [47] , [59] , [60] . These sequences are restricted to arbitrary Z -axis rotations, R z (θ), and arbitrary axis rotations are achieved with standard Euler angle decompositions and additional Hadamard gates. Fortunately, the nature of the Beauregard circuit is such that only arbitrary Z -axis rotations are required (The Quantum Fourier transform can be decomposed into arbitrary Z -axis rotations and CNOTs). We utilize the algorithm of Kliuchnikov et al. [59] , as it has demonstrated the best quantum scaling to date. Each gate in Shor's algorithm is approximated by a sequence of Λ=2 × (3.21log 2 (640 L 4 )−6.93) rotations. The factor of two comes from the fact that the scaling reported in Kliuchnikov et al. [59] is only the number of R z ( π /8) rotations that are needed for approximating an arbitrary rotation. This constitutes approximately half of the sequence, with the additional half consisting mainly of Hadamard operations. Although we assume that the entire sequence consists of R z ( π /8) gates, explicitly constructing fault-tolerant Hadamard operations has only a marginal influence on resources. For further details, see Supplementary Figs S9–S11 and the Supplementary Discussion . How to cite this article: Devitt, S. J. et al. Requirements for fault-tolerant factoring on an atom-optics quantum computer. Nat. Commun. 4:2524 doi: 10.1038/ncomms3524 (2013).